Carrier multiplication in semiconductor nanocrystals detected by energy transfer to organic dye molecules Ever since the first experimental observation of carrier multiplication (CM) in semiconductor nanocrystals (NCs) [1] , this effect has attracted a lot of interest due to its intriguing fundamental physics [2] , [3] , [4] and potential applications in optoelectronic and photovoltaic devices [5] , [6] . Because of the discrete energy levels from the quantum confinement effect and the strong Coulomb interactions between charge carriers, the CM effect is believed to be greatly enhanced in semiconductor NCs as compared with their bulk counterpart materials [7] , [8] . However, the same factors favouring the CM enhancement in NCs also prevent observation of this effect from time-integrated fluorescence measurement by opening a non-radiative Auger decay channel for multiple excitons [9] . For a single NC with two excitons, the biexciton Auger recombination normally occurs on the time scale from tens to hundreds of picoseconds [9] , much shorter than its radiative lifetime [10] , so that the relevant ultrafast optical measurements have to be performed to probe the presence of biexcitons within this relatively short time window. Meanwhile, when a single NC is illuminated with high-energy photons, it is highly possible for it to be ionized with the subsequent formation of charged excitons [11] , which will also undergo the Auger process with a similar time constant to that of the biexcitons. As none of the two commonly used ultrafast optical techniques, that is, pump-probe spectroscopy and time-resolved fluorescence, can directly discriminate between the optical signals coming from multiple and charged excitons [12] , [13] , it is still debated whether the CM efficiency has been truly enhanced in semiconductor NCs [14] , [15] , [16] , [17] . Recently, it has been demonstrated that rigorous stirring of NC solutions with a proper estimation of the photo-charging degree could be a solution to the charged exciton problem [13] . However, it is difficult to remove charged excitons from film NCs using such stirring method, which are closely relevant to the utilization of the CM effect in solid-state devices. It is interesting and urgent to see whether alternative optical methods can be developed to reliably detect the CM effect and estimate its efficiency by excluding false contributions from the charged excitons. Förster resonant or excitation energy transfer (ET) represents an important optical interaction between fluorescent chromophores and has been recently utilized to direct engineered energy flows in semiconductor NC assemblies [18] and to realize single-molecule optoelectronic switches with single NC-dye couples [19] . Unlike direct charge transfer with photo-excited electron or hole moving to the acceptor material [20] , [21] , Förster-type ET proceeds through indirect long-range dipole–dipole interactions that can effectively transfer excitons from the donor to the acceptor chromophores [18] , [19] . 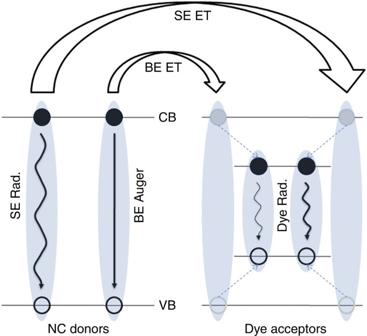Figure 1: Schematic of the ET method for biexciton extraction. Illustration of the competing decay channels of single excitons and biexcitons in the donor NCs and the ET-induced radiative decay of single excitons in the acceptor dyes. A single exciton is represented by the shaded area covering one pair of hollow (hole) and filled (electron) circles. The radiative decay of biexcitons is ignored here, as its lifetime is much longer than the Auger and ET lifetimes. SE, single exciton; BE, biexciton; CB, conduction band; VB, valence band; Rad, radiative decay. Figure 1 shows an ET material system with semiconductor NCs as donors and organic dye molecules as acceptors. Depending on the degree of spectral overlap between the donor emission and acceptor absorption line shapes and their separation distance, the Förster ET lifetime falls at the range of several hundred picoseconds and longer [18] , [22] . When both single excitons and biexcitons are created via CM by high-energy photons in Fig. 1 , it is possible for the biexcitons to take the ET pathway within their Auger lifetime and the acceptor dye fluorescence would be increased accordingly as compared with the case with single excitons alone. Based on the above discussions, we show here that when the excitation photon energy was at ~2.46 times of the CdSe NC energy gap ( E g ), enhanced acceptor dye fluorescence was indeed observed, which could be translated to an average CM efficiency of ~17.1% after the biexciton Auger and ET lifetimes were both measured. Figure 1: Schematic of the ET method for biexciton extraction. Illustration of the competing decay channels of single excitons and biexcitons in the donor NCs and the ET-induced radiative decay of single excitons in the acceptor dyes. A single exciton is represented by the shaded area covering one pair of hollow (hole) and filled (electron) circles. The radiative decay of biexcitons is ignored here, as its lifetime is much longer than the Auger and ET lifetimes. SE, single exciton; BE, biexciton; CB, conduction band; VB, valence band; Rad, radiative decay. Full size image Experimental conditions For the current ET studies, semiconductor CdSe/ZnS NCs (Qdot 525 and Qdot 655 from Invitrogen) and organic Superfluor 680 dyes (same as Alexa Fluor 680 from Invitrogen) were used as the donors and acceptors, respectively, whose solution absorption and emission spectra are shown in Fig. 2 . The aqueous solutions of NCs and dyes, each adjusted to an appropriate concentration, were mixed with the same volume and spin cast onto quartz coverslips to make densely packed solid films. Meanwhile, solid films with only NCs or dyes were also prepared from the above solutions to serve as reference samples. The density of NCs in both the NC-dye mixed and NC-only samples was adjusted to such an extent that the possibility of ET within themselves was minimized, while still keeping a high fluorescence signal. We mainly used a 76-MHz, picosecond 266-nm laser and a continuous wave (CW) 488-nm laser as excitation sources, with their photon energies corresponding to ~2.46 E g (1.97 E g ) and ~1.34 E g (1.08 E g ), respectively, for Qdot 655 (Qdot 525) NCs. The two lasers were both set at the power density of~1 W cm −2 to make the average number ( N ) of single excitons present in each single NC less than 0.1, unless otherwise specified. 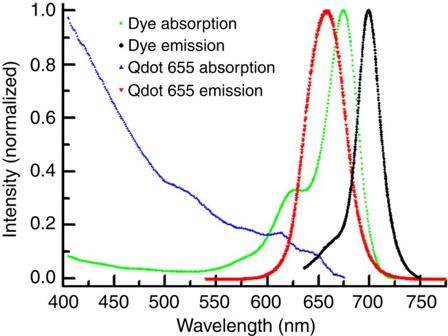Figure 2: Optical characterizations of the solution samples. Normalized absorption and emission spectra of the Qdot 655 NCs and organic dyes measured in solution. Both the absorption and emission spectra are plotted on linear scales. The full absorption spectra of NCs and dyes extending to the wavelengths as short as ~200 nm are plotted inSupplementary Fig. S1a and b, respectively. Figure 2: Optical characterizations of the solution samples. Normalized absorption and emission spectra of the Qdot 655 NCs and organic dyes measured in solution. Both the absorption and emission spectra are plotted on linear scales. The full absorption spectra of NCs and dyes extending to the wavelengths as short as ~200 nm are plotted in Supplementary Fig. S1a and b , respectively. Full size image Enhanced acceptor dye fluorescence With the power density of~1 W cm −2 , the 266-nm laser could not directly excite any detectable fluorescence in the dye-only reference sample, whereas the 488-nm laser induced a very small signal that was about six (thirty) times weaker than the acceptor dye fluorescence excited in the Qdot 525 (Qdot 655) NC-dye mixed sample. In the inset of Fig. 3a , we plot a representative set of photoluminescence (PL) spectra of the Qdot 655 NC-dye mixed sample excited at the same spatial position with the 266 and 488 nm lasers, respectively, which are normalized with respect to the NC emission peaks. As the ET efficiency can be treated as a fixed value within the laser excitation spot and no photons are emitted by biexcitons, the above normalization process guarantees that the same amount of single emissive excitons are initially created in the NCs at these two laser wavelengths. Then the obvious enhancement of the acceptor dye fluorescence by the 266-nm laser strongly suggests that, compared with the 488-nm excitation, it has triggered an additional physical process, which we attribute to the CM effect, in the Qdot 655 NC-dye ET material system. The above conclusion can be further corroborated by the two PL spectra shown in Fig. 3a for Qdot 525 NC-dye mixed sample excited with 266 and 488 nm lasers, respectively, whose photon energies are both below 2 E g of the NCs. The acceptor fluorescence is even a little higher under the 488-nm laser excitation, which is due to a small contribution from the directly excited dye fluorescence discussed earlier in the text. To avoid possible influence of laser characteristics (CW or pulsed) on the PL spectral measurements, we also replaced the CW 488-nm laser by a 76-MHz, picosecond 510-nm laser that has shown similar results as those reported in Fig. 3a . 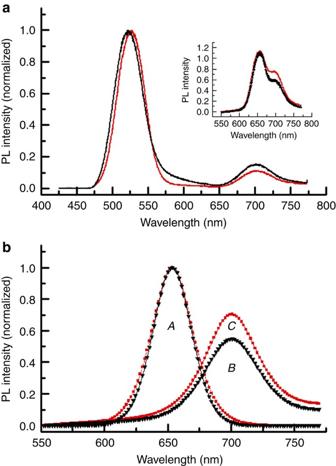Figure 3: PL spectral measurements. (a) PL spectra of the Qdot 525 NC-dye mixed sample excited at 266 nm (red) and 488 nm (black). Inset: PL spectra of the Qdot 655 NC-dye mixed sample excited at 266 nm (red) and 488 nm (black). The two sets of PL spectra were both normalized with respect to the NC emission peaks. (b) Two sets of the NC and dye PL spectra decomposed by Gaussian fits from the two PL spectra shown in the inset of panela. Here,AandBdenote the integrated areas of the NC (excited at 266 nm (red squares) or 488 nm (black triangles)) and dye (excited at 488 nm) PL spectra, respectively, andCis the area difference between the two dye PL spectra excited at 266 and 488 nm, respectively. Figure 3: PL spectral measurements. ( a ) PL spectra of the Qdot 525 NC-dye mixed sample excited at 266 nm (red) and 488 nm (black). Inset: PL spectra of the Qdot 655 NC-dye mixed sample excited at 266 nm (red) and 488 nm (black). The two sets of PL spectra were both normalized with respect to the NC emission peaks. ( b ) Two sets of the NC and dye PL spectra decomposed by Gaussian fits from the two PL spectra shown in the inset of panel a . Here, A and B denote the integrated areas of the NC (excited at 266 nm (red squares) or 488 nm (black triangles)) and dye (excited at 488 nm) PL spectra, respectively, and C is the area difference between the two dye PL spectra excited at 266 and 488 nm, respectively. Full size image Fractional biexciton number In Fig. 3b , the NC and dye PL spectra were decomposed from each of the two PL spectra shown in the inset of Fig. 3a , where A ( B ) represents the integrated area of the NC (dye) PL spectrum excited at 488 nm and C is the area difference between the two dye PL spectra excited at 266 and 488 nm, respectively. If we simply assume that all the single excitons present in the ET material system are eventually converted to photons from either the NCs or dyes, then the ratio of C /( A + B ) should be the fractional number of biexciton transferred to the dyes for each single exciton originally created in the NCs and, in the case of Fig. 3b , yields a value of ~0.075. For a more accurate estimate, parameters such as the PL quantum yields (QYs) and detection efficiencies of the NCs and dyes in the solid films need to be considered, and the number of ~0.075 calculated here only sets a lower limit for the fractional biexciton number (see Methods). Biexciton generation efficiency To evaluate the biexciton generation efficiency in the CM process, we consider the two competing decay channels for biexcitons as depicted in Fig. 1 and divide the fractional biexciton number obtained above by τ 1 /( τ 1 + τ 2 ), in which τ 1 and τ 2 are the biexciton Auger and ET lifetimes, respectively. For the time-resolved fluorescence measurements, we used the 76-MHz, picosecond laser at 266, 400 and 510 nm, respectively, and the corresponding PL decay curves are shown in Fig. 4 . When the 400-nm laser was set at ~25 W cm −2 , the Qdot 655 NC-only reference sample has a single-exponential PL decay curve (black) with a lifetime of ~22.5 ns from the radiative recombination of single excitons [18] . After the power density was increased to ~500 W cm −2 , a fast decay component of ~1.7 ns emerged in the PL decay curve (red), which can be assigned to the biexciton Auger lifetime of the Qdot 655 NCs used here with a radius of ~4.0 nm. In fact, this fast component also appears in the PL decay curve of the Qdot 655 NC-only reference sample excited with much lower power densities ( N <0.1) at 266 nm, which further confirms its Auger origin as reported previously [23] . In Fig. 4 , with the two PL decay curves excited at 266 nm (brown, 50 W cm −2 ) and 400 nm (green, 2.5 kW cm −2 ) displayed together closely, one can clearly see that they match each other very well within the experimental error. To measure the single-exciton ET lifetime, we excited the Qdot 655 NC-dye mixed sample at 510 nm with a power density of ~50 W cm −2 and detected the fluorescence at the blue side of the NC PL spectrum to avoid possible spectral contribution from the dyes. The resulting PL decay curve (blue) is shown in Fig. 4 and a bi-exponential fitting procedure yields an ET lifetime of ~320 ps for single excitons in addition to their radiative lifetime component. In principle, the biexciton ET lifetime should be shorter than the single exciton one, just like in the case of their radiative lifetimes [10] , and here we assume that they are equal to each other for simplicity. Finally, with the two lifetime components of τ 1 =~1.7 ns and τ 2 =~320 ps, we can convert the fractional biexciton number of ~0.075 to the biexciton generation efficiency of ~8.9% for the PL data set shown in Fig. 3b . 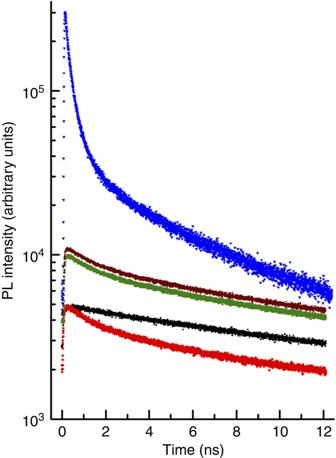Figure 4: Time-resolved measurements. PL decay curves of the Qdot 655 NC-only reference sample excited at 400 nm with the power densities of ~25 W cm−2(black), ~500 W cm−2(red) and 2.5 kW cm−2(green), as well as excited at 266 nm with the power density of 50 W cm−2(brown). PL decay curve of the Qdot 655 NC-dye mixed sample excited at 510 nm with a power density of ~50 W cm−2and detected below 630 nm is also displayed (blue). Except the normalized black and red curves, each of the other three curves was offset to some extent for clarity. Figure 4: Time-resolved measurements. PL decay curves of the Qdot 655 NC-only reference sample excited at 400 nm with the power densities of ~25 W cm −2 (black), ~500 W cm −2 (red) and 2.5 kW cm −2 (green), as well as excited at 266 nm with the power density of 50 W cm −2 (brown). PL decay curve of the Qdot 655 NC-dye mixed sample excited at 510 nm with a power density of ~50 W cm −2 and detected below 630 nm is also displayed (blue). Except the normalized black and red curves, each of the other three curves was offset to some extent for clarity. Full size image Statistics In preparing the NC-dye mixed samples, great care was taken to make densely packed solid films and to put more dye molecules around each single NC for the purpose of receiving extra excitons generated in the CM process. The sample used here represents an optimal one as judged mainly by having the shortest single-exciton ET lifetime. In practice, it is difficult to make a homogeneous film from the spin-casting process and the PL spectra presented in the inset of Fig. 3a were measured in the sample centre, where the chance of seeing more enhanced dye fluorescence is relatively larger. We also made similar PL spectral measurements at ~75 random positions from the film centre to the edge. A histogram for the calculated fractional biexciton numbers from these measurements is depicted in Fig. 5 . The obtained broad distribution is not necessarily caused by the efficiency variation of the CM effect at different sample positions but rather that of the ET process, whose exact lifetime at each position is hard to be resolved due to the limited ~250 ps resolution of our time-resolved system. However, to get a rough estimate, we still use the average ET lifetime of ~320 ps to convert the fractional biexciton numbers in Fig. 5 to the biexciton generation efficiencies, from which an average value of ~17.1% can be deduced. Other ultrafast fluorescence techniques with much higher time resolutions, such as streak camera and optical Kerr gating measurements, would help in the future work to precisely determine the ET lifetimes of solid film samples and thus, narrow down the broad distribution of biexciton generation efficiencies shown in Fig. 5 . 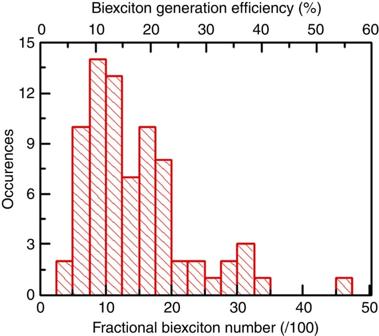Figure 5: Statistics. A histogram for the calculated fractional biexciton numbers at ~75 positions of the Qdot 655 NC-dye mixed sample, together with the converted biexciton generation efficiencies. Figure 5: Statistics. A histogram for the calculated fractional biexciton numbers at ~75 positions of the Qdot 655 NC-dye mixed sample, together with the converted biexciton generation efficiencies. Full size image As reported previously for semiconductor CdSe NCs with an average radius of 3.2 nm ( E g =~2.0 eV), the CM effect was measured with a photon energy threshold of ~2.5 E g , where an extra energy of ~0.5 E g is needed in addition to the energy-conservation-based limit of 2 E g (ref. 24 ). This excess energy, as required by the optical selection rules, is mainly determined by the energy separation between the electron first-excited (1P) and ground (1S) conduction-band states [24] . When the NC radius increases from 3.2 nm to ~4.0 nm for the Qdot 655 NCs used here, the 1P-to-1S energy separation would decrease due to the quantum confinement effect, which naturally explains that the CM process can take place at a slightly smaller photon energy of 2.46 E g in our experiment. Although in the above text we have attributed the enhanced dye fluorescence excited at 266 nm to the generation of biexcitons, it would be necessary to explore whether other mechanisms can enhance the ET efficiency when the excitation photon energy is increased. It has been extensively studied in the literature that carrier relaxation from the higher-lying excited states of CdSe NCs to their band edges is extremely fast, normally on the sub-picosecond timescale [24] . So there should be no change of the ET efficiency from NCs to dye molecules with the 266 nm and 488 nm excitations just based on their different relaxation pathways. However, it is normally the case that the fluorescence QY of semiconductor NCs would decrease with increasing excitation photon energies ( Supplementary Fig. S2 ) [25] . In the case of a single CdSe NC, the fluorescence QY can be roughly calculated from the percentage of the accumulative ‘on’ state time durations within the total measurement time of its PL blinking time trace [26] , [27] . It has been previously reported that the probability of registering longer ‘on’ time periods of PL blinking is reduced when exciting a single CdSe NC with photon energies far exceeding the energy gap [28] . The normalization of the Qdot 655 NC PL intensities in the inset of Fig. 3a sets the condition that the same amount of ‘on’ time durations is collected at the two excitation wavelengths. This implies that, if the 266-nm excitation is associated with a lower QY, longer measurement time has to be used so that more ‘off’ times are accompanied as compared with the 488-nm excitation. Then a critical question is whether these additional ‘off’ time durations contribute to the enhanced dye fluorescence observed here with the 266-nm excitation. In the traditional PL blinking model [11] , the blinking ‘on’ and ‘off’ states of a single NC arise from neutral and charged excitons, respectively. In a charged exciton configuration, it is likely for the single exciton to be transferred to the dye molecules before giving its energy to the extra charge if its Auger lifetime is comparable to the ET one. Although the realization of ET by charged excitons seems to be an equally interesting effect that may be used to extract energy from the ‘off’ state of blinking NCs, we believe this possibility can be reasonably ruled out here based on the following two considerations. First, it was reported that the excitation photon energy has two thresholds at ~1.5 E g and ~3.0 E g , corresponding to the onsets of weak and strong photo-charging of solution NCs, respectively [29] . The 488-nm photon energy is ~1.34 E g for Qdot 655 NCs and ~1.08 E g for Qdot 525 NCs so that the photo-charging probability at this wavelength for both samples is minimal. With the 266-nm excitation, both Qdot 655 (~2.46 E g ) and Qdot 525 (~1.97 E g ) NCs fall within the weak photo-charging regime, with the latter sample having additionally enhanced photo-charging due to the increased leakage of the electronic wave function with reduced size [29] . However, as shown in Fig. 3a for the Qdot 525 NC-dye ET system, the fact that no enhanced acceptor fluorescence was observed with the 266-nm excitation strongly supports that PL blinking ‘off’ states, or charged excitons, only have a negligible role for the enhanced ET process in the inset of Fig. 3a . Second, it was recently reported [30] that the ‘off’ state fluorescence QY of single CdSe NCs can be ~10 (~100) times less than that of the biexciton (neutral exciton). One proposed mechanism was that the PL blinking ‘off’ state could be caused by the temporary opening of an extremely fast decay pathway of neutral excitons so that a single NC is not necessarily charged [31] , [32] , [33] . An alternative mechanism was that multiplely charged excitons are involved in the PL blinking ‘off’ state with a non-radiative decay lifetime that is too fast to be explained by the Auger process with singly charged excitons [30] . The above observation agrees well with the experimental results obtained from our PL blinking studies of single Qdot 655 NCs with an ‘on’/’off’ intensity ratio of >100 ( Supplementary Fig. S3 ). Similarly, we observed a ratio of >40 between the ET efficiencies from the ‘on’ and ‘off’ states of a single Qdot 655 NC to its surrounding dyes, which will be reported elsewhere. If the PL blinking ‘off’ state is really caused by charged excitons, the above ratio confirms that their contribution to the enhanced dye fluorescence in the inset of Fig. 3a is trivial (see Methods). Finally, we would like to elaborate on the 1.7-ns lifetime of biexciton Auger recombination shown in Fig. 4 and also confirmed from an ultrafast transient absorption measurement ( Supplementary Fig. S4 ). The structural properties of the NC sample used here have been previously characterized with a radius of ~4.0 nm and an aspect ratio of ~1.8 [34] , [35] . These NCs can be treated either as spherical dots or elongated rods but, in both cases, will have a biexciton Auger lifetime of ~400 ps according to its volume dependence reported before [36] . Meanwhile, exactly the same NCs, together with the ‘giant’ CdSe/CdS NCs, are the only two CdSe samples that have shown efficient biexciton fluorescence on the single NC level [35] , [37] . Specifically, a QY of ~80% was measured for the biexciton fluorescence of this sample at ~140 K [35] , which implies a great suppression of the non-radiative Auger process, so that its lifetime should deviate significantly from the value predicted by the volume dependence [36] . The 1.7-ns lifetime measured here seems to reflect the fact that the Auger suppression might be elevated at room temperature but is still relatively strong. It should be pointed out that this 1.7-ns lifetime component cannot be associated solely with biexcitons and a significant portion of it may come from the charged exciton decay, as deduced from the transient absorption measurement ( Supplementary Fig. S4 ). In conclusion, we have demonstrated that biexcitons generated in semiconductor NCs from the CM effect can be extracted to the organic dye molecules via an efficient ET process, resulting in an enhanced acceptor fluorescence with the excitation of high-energy photons. The introduction of ET to the current CM studies has not only provided a novel way to unambiguously confirm its existence in semiconductor NCs but also has the potential to precisely estimate its efficiency if an appropriate model can be developed. Under certain simplified assumptions, an average biexciton generation efficiency of ~17.1% was determined in semiconductor CdSe NCs when the excitation photon energy is ~2.46 times of their energy gap. We believe that the extended storage of multiple excitons from the NC Auger lifetime to the acceptor radiative one in a well-designed ET material system would mitigate the stringent requirement of fast charge separations and thus, facilitate the utilization of CM effect in future solar cell technologies. The Förster resonant ET method used here is similar to the space-separated quantum cutting (SSQC) approach reported before [25] , [38] in terms of extracting extra excitation energies from the donor to the acceptor materials. In the SSQC case, the relaxation energies of the photo-excited carriers above the energy gap of Si NCs can be effectively transferred to the doped Er 3+ ions or nearby Si NCs with subsequently enhanced PL QY [38] . Because of the Auger-assisted nature of SSQC, two excitons can be simultaneously prepared in two separate Si NCs once the excitation photon energy is tuned to just above 2 E g (ref. 25 ). In our case, two excitons are created within and transferred from the same CdSe NC to the nearby dye molecules through the Förster-type dipole–dipole interactions, and an extra energy above 2 E g is normally needed to trigger the CM process. It would be interesting in the future work to compare the multiple exciton generation efficiencies of the above two methods and even combine them in a suitable ET material system for the harvesting of more high-energy photons from the solar spectrum. Optical measurements The 800-nm output of a 76-MHz, picosecond Ti:sapphire laser (Mira HP, Coherent Inc.) was used to get the wavelengths of 266, 400 and 510 nm from the THG (third harmonic generation), SHG (second harmonic generation) and OPO (optical parametric oscillation) processes, respectively. For the PL spectral measurements, the excitation laser beam was focused onto the sample surface with a diameter of ~100 μm at an incident angle of ~45° relative to the surface normal direction. The sample PL was collected vertically from the surface by a × 50 microscope objective and sent through a 0.5-m spectrometer to a charge-coupled-device camera. For the time-resolved PL decay measurements, the ultrafast laser beam was focused on the sample surface by a × 60 microscope objective with a diameter of ~100 μm. The sample PL was collected by the same objective and sent to an avalanche photodiode in the time-correlated single photon-counting system with a time resolution of ~250 ps. All the measurements were performed at room temperature. Charged exciton contribution to enhanced dye fluorescence In Fig. 3b , A + B represents the total number of neutral excitons generated in the ET system ( A and B are the numbers of neutral excitons staying in the NCs and transferred to the dyes, respectively), and C is the number of excitons additionally received by the dyes from ET of charged excitons and/or biexcitons. The ET efficiency of charged excitons can be estimated to be B /[40( A + B )] using the neutral exciton ET efficiency of B /( A + B ) and the ET efficiency ratio of ~40 between the neutral and charged excitons discussed in the text. As measured by Padilha et al. [29] , the fraction of charged NCs in a solution sample reaches a value of ~0.2 when the excitation photon energy is ~4.5 E g in the strong photo-charging regime. As the 488-nm photon energy used here for Qdot 655 NCs (~1.34 E g ) is below the weak photo-charging threshold of ~1.5 E g , we can assume that NCs excited at this wavelength is free of charged excitons. Meanwhile, for the 266-nm laser with a photon energy of ~2.46 E g close to the strong photo-charging threshold of ~3.0 E g , we can assume an upper limit of ~0.2 for the fraction of charged NCs. For A + B neutral excitons created at both 488 nm and 266 nm, the number of charged excitons associated with the latter excitation should be ( A + B )/4. This number, when multiplied by the ET efficiency of B /[40( A + B )] for charged excitons, results in a value of B /160=~0.16 (taking B =26.11 from Fig. 3b ) for extra excitons transferred to the acceptor dyes with the 266-nm excitation, which is significantly smaller than the experimentally measured value of C =4.90. If we take the fact that the NCs might be already charged at 488 nm, the charged exciton contribution to the enhanced dye fluorescence at 266 nm would be even smaller than the ~0.16 value. With the measured values of ~100 and ~40 for the PL QY and ET efficiency ratios between neutral and charged excitons, the contribution of photo-charging effect to the enhanced dye fluorescence can be evaluated in an alternative way by simply comparing the relative changes in the NC and dye PL intensities excited at the two laser wavelengths. We can assume that the ET efficiency of NC neutral excitons is η and a fixed amount of photons ( I ) is absorbed by the NCs. At 488 nm, the PL intensities are I (1− η ) and Iη for the NCs and dyes, respectively, leading to a PL intensity ratio of (1− η )/ η . At 266 nm, the PL intensity of NCs has contributions from both neutral and charged excitons, which are 0.8 I (1− η ) and 0.2 I (1− η /40)/100, respectively. At this wavelength, the ET-induced dye PL intensities from neutral and charged excitons are 0.8 Iη and 0.2 Iη /40, respectively. Then the PL intensity ratio between NCs and dyes at 266 nm would be [0.8(1− η )+0.2(1− η /40)/100]/[0.8 η +0.2 η /40], which can be further reduced to (1− η )/ η , as the second terms in both the numerator and denominator are significantly smaller than their respective first ones. Based on the above calculations, it can be again confirmed that the relative changes in the NC and the ET-induced dye PL intensities excited at the two wavelengths are approximately the same and not influenced by the photo-charging effect. Calculations of the fractional biexciton number We define α ( α′ ) and β ( β′ ) as the fluorescence QY and detection efficiency of the NC (dye) excitons, respectively. From Fig. 3b of the manuscript, A /( αβ )+ B /( α′β′ ) should be the total number of neutral excitons generated in the NCs, and C /( α′β′ ) the number of biexcitons transferred to dyes. Then [ C /( α′β′ )]/[ A /( αβ )+ B /( α′β′ )] would be the fractional number of biexciton transferred to the dyes for each neutral exciton originally created in the NCs. As the detector, grating and mirrors used in our experiment have almost flat light-responsive curves within the wavelength range of the NC and dye PL (that is, β = β′ ), the fractional biexciton number becomes C /[ A ( α′ / α )+ B ] and further to C /( Aα′ + B ) when assuming α =1 for neutral excitons. In practice, α′ is always smaller than 1 so that the fractional biexciton number calculated in the text using α′ =1 should only be a lower limit of the real one. How to cite this article: Xiao, J. et al. Carrier multiplication in semiconductor nanocrystals detected by energy transfer to organic dye molecules. Nat. Commun. 3:1170 doi: 10.1038/ncomms2183 (2012).